Electroneutrality breakdown and specific ion effects in nanoconfined aqueous electrolytes observed by NMR Ion distribution in aqueous electrolytes near the interface plays a critical role in electrochemical, biological and colloidal systems, and is expected to be particularly significant inside nanoconfined regions. Electroneutrality of the total charge inside nanoconfined regions is commonly assumed a priori in solving ion distribution of aqueous electrolytes nanoconfined by uncharged hydrophobic surfaces with no direct experimental validation. Here, we use a quantitative nuclear magnetic resonance approach to investigate the properties of aqueous electrolytes nanoconfined in graphitic-like nanoporous carbon. Substantial electroneutrality breakdown in nanoconfined regions and very asymmetric responses of cations and anions to the charging of nanoconfining surfaces are observed. The electroneutrality breakdown is shown to depend strongly on the propensity of anions towards the water-carbon interface and such ion-specific response follows, generally, the anion ranking of the Hofmeister series. The experimental observations are further supported by numerical evaluation using the generalized Poisson–Boltzmann equation. Electric double layer near the interface is of fundamental importance in various applications ranging from electrochemistry [1] and electrophoresis [2] , to colloidal particles assembly [3] and nanofluidics [4] . The neutrality of the total charge is an important condition in deriving the ion distribution near the interface in the electric double layer theory. For an uncharged hydrophobic surface such as the water/air interface, positive and negative ions can still be separated in the interfacial region (~10 Å) due to different propensities towards the interface between the cations and anions [5] , [6] , [7] , [8] ; such effect is called specific ion effect [9] , [10] , [11] , [12] , [13] since it is driven by non-electrostatic interactions that vary significantly between different ions even for ions with the same electrovalency (for example, F − and I − ). In the scenario of aqueous electrolytes confined by hydrophobic surfaces where the pore size is comparable in size to the interfacial region determined by the specific ion effect, a natural question raised is how the tendency of charge separation near the interface reconciles with electroneutrality inside nanoconfined regions. Could electroneutrality of the total charge in fact be violated substantially inside nanoconfined regions driven by the specific ion effect? Theoretical studies nearly always take the total charge neutrality inside nanoconfined regions for granted and experimental evaluation of electroneutrality inside nanoconfined regions is lacking. Such evaluation could contribute significantly to our understanding of some very important processes such as energy storage in supercapacitor [14] , ion transport through nanochannels [15] and ionic processes in proteins [9] . Nanoporous carbon with graphitic-like internal surfaces provides an ideal model system for investigating the electroneutrality in nanoconfined aqueous electrolytes using nuclear magnetic resonance (NMR). Previous studies showed that fluid inside carbon nanopores exhibits a different NMR chemical shift from that outside the nanopores due to the ring current effect, which gives rise to a nucleus-independent chemical shift [16] , [17] , [18] , [19] , [20] . This shift provides a clear NMR marker for selectively and quantitatively monitoring the electrolyte inside nanometer-sized regions confined by hydrophobic graphitic-like carbon surfaces. It provides an excellent tool for determining quantitatively the cation and anion concentrations inside nanopores. Ions, especially anions, can be ordered by their influence on a vast variety of specific ion effects, called the Hofmeister series [9] , [12] , [21] . A typical ranking is SO 4 2− <F − <Cl − <Br − <NO 3 − <I − <BF 4 − <ClO 4 − for some anions with increasing protein solubility in aqueous electrolytes to the right side (often referred to as the chaotropic side) [12] . Evaluating the electroneutrality with systematic change of anions according to the Hofmeister series provides another avenue for revealing the potential electroneutrality breakdown caused by the ion-specific interfacial effect. Here we report such a quantitative NMR study of the ion concentrations in nanoconfined aqueous electrolytes. Hydrophobic graphitic-like porous carbon is used as a model system to provide the nanoconfinement. Direct experimental evidence is observed for a significant electroneutrality breakdown of the total charge inside nanometer-sized regions even when the carbon material is uncharged. Interfacial specific ion effects and ion–ion correlations are shown to play crucial roles in determining the degree of electroneutrality breakdown inside nanopores. The importance of the specific ion interfacial effect is further revealed by the asymmetric and nonlinear responses of cation and anion concentrations to the external charging of the nanoconfining carbon walls. Such information is obtained using a charge-controlling device built into the NMR probe. The experimental results are further validated by a numerical calculation using the generalized Poisson–Boltzmann equation in nanopores, demonstrating that specific ion interfacial effect can indeed dominate the electrostatic interactions leading to the breakdown of electroneutrality inside nanoconfined regions. Electroneutrality breakdown in nanoconfinement A high-quality nanoporous carbon derived from polymer polyetheretherketone (PEEK) [22] , [23] is used to provide the hydrophobic nanoconfinement in this work (see Methods). The activated carbon sample is designated as P-40 and the average pore size is 0.9 nm from wall surface to wall surface assuming a slit-shaped pore (1.2 nm from carbon centre to carbon centre) according to the previous study [17] . Unless specified, all results discussed here refer to that obtained using P-40. However, activated carbon with pore size of 1.9 nm (carbon to carbon centres), labelled P-92, was also used in the current study and will be mentioned as well. The capability of NMR approach to selectively and quantitatively study nanoconfined fluids is demonstrated in Fig. 1a where the 1 H, 19 F and 23 Na static NMR spectra of NaBF 4 electrolyte injected into P-40 are shown (see Methods). All spectra consist of two peaks. The peak centred at 0 p.p.m., chosen as the reference, comes from electrolyte outside the nanopores while the peak centred at −7 p.p.m. is from electrolyte inside nanopores [16] . All the three nuclei show the same chemical shift at −7 p.p.m. because the shift is completely determined by the nucleus-independent chemical shift effect. 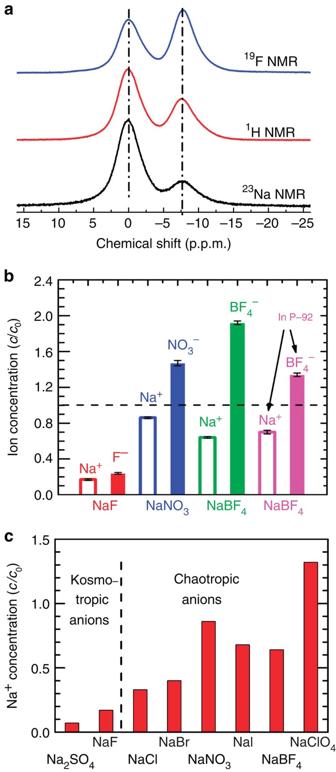Figure 1: Ion concentrationsc/c0in uncharged P-40 carbon nanopores. (a)19F,1H and23Na static NMR spectra of 30 μl 1 mol kg−1NaBF4electrolyte in 20 mg P-40. The peak on the left is chosen as the reference (0 p.p.m.) and the right peak is centred at −7 p.p.m. for all the three nuclei due to nucleus-independent chemical shift. (b) Cation and anion concentrations of NaF, NaNO3and NaBF4electrolytes inside P-40 nanopores. NaBF4electrolyte in a larger pore size sample P-92 is also shown for comparison. (c) Na+concentration inside the nanopores for different sodium salt electrolytes plotted in the sequence of the anionic Hofmeister series. Figure 1: Ion concentrations c / c 0 in uncharged P-40 carbon nanopores. ( a ) 19 F, 1 H and 23 Na static NMR spectra of 30 μl 1 mol kg −1 NaBF 4 electrolyte in 20 mg P-40. The peak on the left is chosen as the reference (0 p.p.m.) and the right peak is centred at −7 p.p.m. for all the three nuclei due to nucleus-independent chemical shift. ( b ) Cation and anion concentrations of NaF, NaNO 3 and NaBF 4 electrolytes inside P-40 nanopores. NaBF 4 electrolyte in a larger pore size sample P-92 is also shown for comparison. ( c ) Na + concentration inside the nanopores for different sodium salt electrolytes plotted in the sequence of the anionic Hofmeister series. Full size image Since the NMR signal is proportional to the number of spins, numbers of cations outside and inside the nanopores can be determined by the 23 Na peak intensities at 0 and −7 p.p.m., respectively. Similarly, numbers of BF 4 − anions and water molecules outside and inside nanopores can be determined from the corresponding peak intensities of the 19 F and 1 H NMR spectra, respectively. From these numbers the cation and anion average concentrations inside the nanopores can be determined (see Methods). Fig. 1b shows the normalized ion concentrations, c / c 0 , where c is the average ion concentration in nanopores and c 0 is the injected electrolyte concentration (1 mol kg −1 except for NaF 0.8 mol kg −1 due to its lower water solubility), for NaF, NaNO 3 , NaBF 4 electrolytes in P-40 and NaBF 4 electrolyte in P-92. One of the surprising phenomena revealed by measurements shown in Fig. 1b is the drastic concentration difference between cations and anions, particularly significant in nanoconfined aqueous electrolytes of NaNO 3 and NaBF 4 . The concentration inside nanopores is c / c 0 =1.92 for BF 4 − and c / c 0 =0.64 for Na + . In the larger pore P-92 sample, the concentration inside nanopores is c / c 0 =1.34 for BF 4 − and c / c 0 =0.70 for Na + . The anomalous concentration difference is a strong indication of the electroneutrality breakdown of the total charge inside the nanopores. As expected, the electroneutrality breakdown is less in the larger pore P-92 sample but it is, nevertheless, still very significant. The possibility that the electrolyte neutrality might be maintained by other ions such as H + , OH − or trace impurities can be ruled out in the current experimental approach. Take NaF electrolyte in P-40 as an example to estimate the amount of H + and OH − . The PEEK-derived activated carbon is of high quality and contains very few surface functional groups [23] , [24] that do not produce H + or OH − . So we can conclude that all the H + and OH − in this system are from the dissociation of water (depending on the point of zero charge and pH, the activated carbon can be positively or negatively charged, but the source of the charge still comes from water dissociation). Since only limited electrolyte is injected into the activated carbon, the electrolyte amount in the intergranular space is only about three times that inside carbon nanopores. The intergranular electrolyte pH is measured to be 10 in the slurry. Therefore the net charge due to H + or OH − inside carbon nanopores is at most 3 × 10 −4 mol kg −1 , which is negligible compared with the ion concentration inside nanopores (Na + 0.17 mol kg −1 , F − 0.24 mol kg −1 ). Similar estimate can be applied to other ions and the trace impurities (<1%) in the as purchased chemicals. Even if the impurities are all segregated into the nanopores, the maximum concentration is at most four times the impurity concentration in the bulk electrolyte. This would give rise to an estimated impurity concentration of 0.04 mol kg −1 , which is insignificant compared with the charge imbalance on the order of 0.5 mol kg −1 . This shows that the electroneutrality breakdown of the total charge inside carbon nanopores is an intrinsic property of nanoconfined aqueous electrolytes in this system. Specific ion effects on ion concentrations Another intriguing phenomenon beyond the electroneutrality breakdown revealed by the data in Fig. 1b is the strong influence of anions on Na + concentration. Although the experiments are carried out with similar electrolyte concentrations and electrolyte/carbon ratios, the Na + concentrations vary significantly among the different electrolytes. Na + concentration for NaF electrolyte in nanopores is highly suppressed while that for NaNO 3 is close to the injected electrolyte concentration. It is interesting to note that the anion concentration increases in the order F − <NO 3 − <BF 4 − with F − concentration being also highly suppressed in the nanopores while NO 3 − and BF 4 − concentrations being greatly enhanced. The F − <NO 3 − <BF 4 − ranking based on their concentrations is fully consistent with the ranking of the Hofmeister series where the anions are known to have different propensities for a hydrophobic surface [9] . Systematic testing on a series of sodium salt electrolytes whose anions are chosen from the Hofmeister series SO 4 2− <F − <Cl − <Br − <NO 3 − <I − <BF 4 − <ClO 4 − provides more insights into the anion-dependent Na + concentrations inside the nanopores. The normalized average Na + cation concentration c / c 0 for the sodium salt series is shown in Fig. 1c . Na + concentration inside nanopores increases gradually from Na 2 SO 4 to NaClO 4 following the anion Hofmeister series with NaNO 3 being a clear exception (and slightly for NaI). It is of note that Na + concentration inside nanopores is highly suppressed to c / c 0 <0.2 for Na 2 SO 4 and NaF, <0.4 for NaCl and NaBr, and <0.7 for NaI and NaBF 4 . Even though I − and BF 4 − are ranked to the right side (the chaotropic side) of NO 3 − in the Hofmeister series, c / c 0 =0.86 for NaNO 3 is significantly higher than that of NaI and NaBF 4 . It is also of note that unlike other electrolytes, Na + concentration for NaClO 4 in nanopores is substantially enhanced ( c / c 0 =1.32) rather than suppressed. Because limited amount of electrolyte is added to the sample, Na + concentration outside the nanopores also differs from c 0 . The Na + concentration in nanopores normalized by that outside the nanopores shows slightly different values from c / c 0 but maintains the same trend of Na + concentration increase including the NaNO 3 anomaly. The strongly anion-dependent Na + concentration inside carbon nanopores revealed by the quantitative NMR analysis demonstrates the intriguing interplay between cations and anions. Na + is a strongly hydrated cation with hydration free energy of −87 kcal mol −1 , hydration number of 5–6 in the first hydration shell [25] , [26] , and no propensity for the interface [10] . In fact, strong hydration leads to a free-energy barrier of several k B T ( T =300 K) or higher for Na + ions to enter the hydrophobic nanopore with diameter <2 nm (ref. 27 ). This is clearly reflected by the low value of c / c 0 <0.2 for Na + in NaF. Theory predicts F − <Cl − <I − to be the ranking based on their propensity for the interface [10] . This trend is expected to hold for most anions in the Hofmeister series where the hydration enthalpy becomes less negative towards the chaotropic side of the series [28] . In nanopore confinement, the different ion–water and ion-surface interactions among those anions lead to the differences in Na + cation concentrations. Specific ion effects are ubiquitous in electrochemical and biological systems [9] , [10] , [12] , [29] . It is very fascinating that very different effects such as the bulk effect of viscosity [30] , [31] and interfacial effect such as surface tension [21] , [32] all follow the same trend as described by the Hofmeister series. The common thread linking all these effects is hydration and the unique properties of water. It was suggested that when ion–water interaction is stronger than water–water interaction the Jones–Dole coefficient B is positive (for example, F − ), whereas it is negative when water–water interaction is stronger than ion–water interaction (for example, BF 4 − and NO 3 − ). In fact, the sign change in B (positive to negative) is correlated with our observation where anion concentration changes from being suppressed to being enhanced. This indicates that the relative strength of ion–water versus water–water interaction also plays a dominant role in the specific ion effects in nanoconfinement by hydrophobic surfaces. Numerical calculation More insight into the anion’s influence on Na + concentration can be gained by looking at the various factors determining the ion distribution near the interface. The ion distribution for ion i with valency z i is given by [32] , [33] where e is the elementary charge, Λ i is the de Broglie thermal wavelength of ion i , μ i is the chemical potential of ion i , ψ ( x ) is the local electrostatic potential at the location x inside nanopores, is the ion-surface potential that depends on the ion-specific propensity for the interface [33] , [34] and corr i ( x ) is the free-energy contribution from ion–ion correlations. For 1 mol L −1 monovalent ions, the electrostatic correlation [35] is of minor importance and corr i ( x ) is dominated by the non-electrostatic excluded-volume interactions, which require molecular scale structural information to obtain, such as via theory and molecular dynamics simulations [33] . corr i ( x ) depends on both the ion-specific short-ranged pair potential and the ion concentrations, which are implicitly affected by the electrostatic potential ψ ( x ). The ion concentration measured by NMR is the averaged value over the pore width . Although ion-surface potential is generally position dependent and has an oscillatory character [34] , [36] , it is expected that the mean potential for anions, defined by , ranks according to the Hofmeister series in P-40 nanopores. As such, a larger value for the more chaotropic anion would lead to a higher anion concentration and that would attract more Na + counterions into nanopores electrostatically. Of course, this argument does not take into considerations of the ion–ion correlations (that is, corr i ( x )=0). Numerical calculation using the generalized Poisson–Boltzmann equation in a 1D planar pore is carried out to reveal the mechanism of the electroneutrality breakdown in nanoconfined aqueous electrolytes (see Methods). Since the ion-surface potential [34] , [37] and ion–ion correlation functions [36] , [38] , [39] from molecular dynamics simulation are not available for our system, we ignore the ion–ion correlations at this moment and use a simplified ion-surface interactions potential [40] . Here x is the distance from the ion centre to the confining surface ( x >x min , x min is the cutoff distance from ion centre to the surface, which defined the Helmholtz plane); B i characterizes the strength of the ion-specific interfacial interaction whose value is about few k B T near the surface [41] . To focus on the effects of ion-specific interactions, the electrostatic interaction with its image charge is not accounted here since it is not ion-specific. Similar to the Jones–Dole coefficient B, positive B i will be used for strongly hydrated ions (for example, F − and Na + ), which are repelled from the surface, whereas weakly hydrated ions (for example, BF 4 − and NO 3 − ) will have negative B i indicating their affinity to the surface. Because the boundary condition on the metal plate is unknown (even though the net charge on the metal plate is 0, we could not assume the surface charge is 0 because the inner surface and outer surface may carry induced charges of an equal amount but opposite signs), electrostatic potentials both inside and outside the nanopore need to be solved simultaneously to find the ion distribution inside nanopores (see Methods). Ion distribution in a 1 nm 1D planar pore is illustrated in Fig. 2b . In this calculation we use B i value −58 × 10 −50 J m 3 and 46 × 10 −50 J m 3 (about 5 k B T at 0.3 nm from the surface) for anions and cations, respectively. Anions are preferentially adsorbed on the surface because an attractive potential is chosen, whereas cations are repelled from the surface. The average anion concentration in the nanopore is much higher than that of cation, indicating an electroneutrality breakdown of the total nanoconfined charge. Clearly, the ion-surface interaction is responsible for such electroneutrality breakdown. If only Columbic interaction is considered as in the Gouy–Chapman theory, that is, , bulk concentration will be obtained in nanopores and the total charge is neutral. 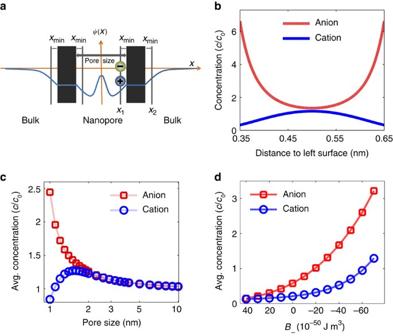Figure 2: Numerical calculation using generalized Poisson–Boltzmann equation. (a) Two conducting metal plates are immersed in 1 M 1:1 electrolyte to simulate the 1D planar carbon nanopore with pore sized. The pore centre is set asx=0.xminis defined as the closest distance that the ions can approach the surface. (b) Ion distribution in 1-nm pores forB+=46 × 10−50J m3,B−=−58 × 10−50J m3. (c) Average ion concentration in nanopores versus pore size. (d) Average ion concentration in nanopores versus the parameterB−. The parameterB+=46 × 10−50J m3is fixed. Figure 2: Numerical calculation using generalized Poisson–Boltzmann equation. ( a ) Two conducting metal plates are immersed in 1 M 1:1 electrolyte to simulate the 1D planar carbon nanopore with pore size d . The pore centre is set as x =0. x min is defined as the closest distance that the ions can approach the surface. ( b ) Ion distribution in 1-nm pores for B + =46 × 10 −50 J m 3 , B − =−58 × 10 −50 J m 3 . ( c ) Average ion concentration in nanopores versus pore size. ( d ) Average ion concentration in nanopores versus the parameter B − . The parameter B + =46 × 10 −50 J m 3 is fixed. Full size image The ion concentrations depend on the pore size and the strength of the anion–surface interactions. The average ion concentration versus pore size is shown in Fig. 2c . The B i values are the same as in Fig. 2b . The electroneutrality breakdown is prominent only when the pore size is <2 nm. As the pore size increases, the concentration difference between the cations and anions disappears and both the ion concentrations approach that of the bulk value. Figure 2d shows the average ion concentration versus B − , demonstrating the specific ion effects on the extent of the electroneutrality breakdown in 1 nm pores. Here B + is fixed at 46 × 10 −50 J m 3 while B − varies from 40 × 10 −50 to −70 × 10 −50 J m 3 to represent the increased ion propensity for the interface. The average anion concentration increases as expected when B − becomes more negative. Although B + is kept unchanged, cation concentration also increases because of the increased electrostatic attraction to the anions. The electroneutrality breakdown is more prominent as the propensity difference between cations and anions grows. It is of note that the numerical calculation here shows a monotonic increase of the cation concentration, which could not explain the anomaly of high Na + concentration in nanoconfined NaNO 3 electrolyte. This is mainly because ion–ion correlations are not included in this calculation. The ion–ion correlations based on electrostatic and ion-specific interactions are predicted to be of crucial importance in nanoconfined electrolytes [33] , [36] , [38] , [42] , [43] . Although the preferentially adsorbed anions in the nanopores could attract Na + cations via electrostatic interactions as demonstrated by both the experiments and the simulation, the higher Na + concentration associated with NaNO 3 electrolyte is not due to the anomalous interfacial affinity of NO 3 − since its concentration is consistent with the ranking of the Hofmeister series, that is, lower than the BF 4 − concentration ( Fig. 1b ). Clearly, specific ion–ion correlations must be invoked to explain the abnormal Na + concentration in NaNO 3 . Correlations of Na + with NO 3 − appear to be stronger than that with I − and BF 4 − , suggesting a more negative mean correlation , defined by , for Na + inside the nanopores. It is interesting to note that the formation of solvent-separated Na + and NO 3 − ion pairs in bulk electrolyte has been recognized by both computational and experimental studies [44] , [45] . The formation of solvent-separated Na + and ClO 4 − ion pairs was also found in bulk electrolyte [46] . Such molecular scale ion–ion correlations could become more significant at the interface and in nanoconfined environment giving rise to the observed anomaly in the Na + concentration of NaNO 3 and the substantially enhanced Na + concentration in NaClO 4 aqueous electrolyte. Ion concentrations in charged nanopores To further demonstrate how the non-electrostatic specific ion effects including ion–ion correlations dominate the electrostatic interactions inside the nanopores and lead to the intriguing electroneutrality breakdown, ion concentrations versus confining wall surface charging is measured with the in situ NMR [47] , [48] , [49] . As a model system to investigate electrolyte properties under hydrophobic nanoconfinement, the electric conducting property of activated carbon is an additional benefit that allows fine control of the surface charge to tune the electrostatic interactions. This is achieved by incorporating a device similar to a supercapacitor [14] , [50] , [51] into an NMR probe (see Methods). As illustrated in Fig. 3a , two electrodes made of P-40 are separated by a glass fibre and immersed in an aqueous electrolyte. Voltage can be applied between the two electrodes to change the surface charge while NMR spectrum is acquired in situ . The ion concentration inside the nanopores versus charging voltage is measured for a single electrode while the other one is covered with a copper foil to shield the radio frequency pulse and signal. 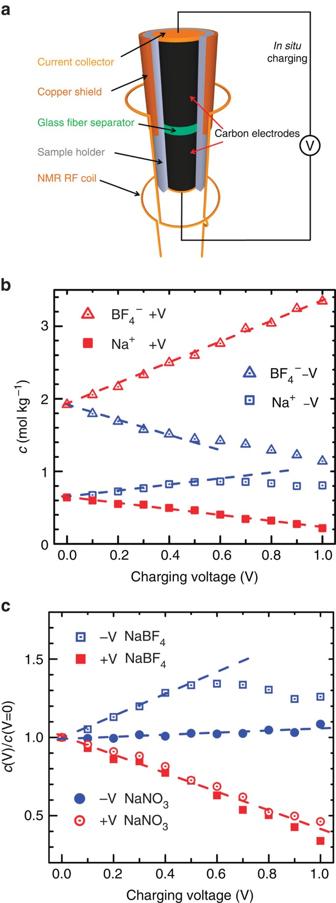Figure 3: Ion concentrations in charged P-40 nanopores versus charging voltage. (a) Illustration of the device built into an NMR probe for controlling P-40 surface charging. The device is comprised of two P-40 electrodes immersed in electrolyte and separated by a glass fibre (similar to a supercapacitor). Voltage is applied between the two electrodes such that one electrode is positively charged and the other one is negatively charged. One electrode is covered by copper foil to enable single-electrode NMR measurements. (b) Nanoconfined ion concentrations for 1 mol kg−1NaBF4electrolyte in P-40 versus charging voltage. (c) Comparison of Na+concentrationsc(V)/c(0) between NaBF4and NaNO3electrolytes versus charging voltage. Figure 3: Ion concentrations in charged P-40 nanopores versus charging voltage. ( a ) Illustration of the device built into an NMR probe for controlling P-40 surface charging. The device is comprised of two P-40 electrodes immersed in electrolyte and separated by a glass fibre (similar to a supercapacitor). Voltage is applied between the two electrodes such that one electrode is positively charged and the other one is negatively charged. One electrode is covered by copper foil to enable single-electrode NMR measurements. ( b ) Nanoconfined ion concentrations for 1 mol kg −1 NaBF 4 electrolyte in P-40 versus charging voltage. ( c ) Comparison of Na + concentrations c (V)/ c (0) between NaBF 4 and NaNO 3 electrolytes versus charging voltage. Full size image Figure 3b shows the ion concentrations inside P-40 nanopores versus charging voltage for NaBF 4 electrolyte measured by 19 F and 23 Na NMR. On positive charging (+V), both Na + and BF 4 − concentrations respond linearly with the charging voltage. The influence of the non-electrostatic interactions is reflected on the huge initial concentration difference at 0 V. Because the surface is already crowded with anions at 0 V, further positive charging is unlikely to bring in more anions to the surface where non-electrostatic interactions are dominant. Therefore, such a linear behaviour is expected when the ion concentration change is mainly due to ions away from the interface and is affected by the change of electrostatic interactions [33] . In contrast, both Na + and BF 4 − exhibit nonlinear behaviour on negative charging (−V). Na + concentration increases with voltage from 0 to 0.6 V but then starts to decrease with further negative charging. Concomitantly, the initial linear decrease of BF 4 − concentration levels off beyond 0.6 V. The nonlinear behaviour, particularly the unexpected Na + concentration decrease with negative charging beyond 0.6 V, demonstrates the competing effect between the ion–ion correlations and the ion-surface electrostatic interactions. The attractive Coulomb interaction between Na + and the negatively charged surface tends to bring Na + into the nanopores, whereas the decreased BF 4 − concentration favours the dragging of Na + out of the nanopores. When the latter effect dominates, the Na + concentration can actually decrease with further negative charging as observed in Fig. 3b . It is also interesting to note that even at 1.0 V charging, the BF 4 − concentration in nanopores is still higher than that of Na + , demonstrating the strong ion-surface attractions that overcomes the enormous Coulombic forces due to the net charge in the nanopores and the repulsion between the anions and the negative charged surface. The influence of anions on the cation’s behaviour via ion–ion correlations is evidenced by comparing Na + behaviours between NaBF 4 and NaNO 3 electrolytes shown in Fig. 3c . For the convenience of comparison, the concentration has been normalized by their respective value at 0 V. On positive charging, Na + concentrations in both NaBF 4 and NaNO 3 decrease linearly because they are mainly affected by the change in electrostatic interactions. However, drastically different behaviours are observed on negative charging: while response of Na + in NaBF 4 electrolyte first increases then decreases, the Na + concentration for NaNO 3 almost does not change with charging voltage, indicating that the correlation between Na + and NO 3 − is stronger than that in NaBF 4 . The Coulombic attraction on the cations by the negatively charged surface is completely compensated by the ion–ion correlations that drags Na + out of the nanopores when the anions are repelled from the nanopores. Charge separation is a critical step in many biological processes and important device applications. For instance, when the confining walls of a nanochannel carry certain preset surface charge, complete screening inside the nanochannel cannot be accomplished by the counter ions when the nanopore size becomes comparable to the Debye length. A potential difference, the Donnan potential [52] , [53] , [54] , between the inside and outside of the nanochannel is established and this can have a strong influence on ionic transport and the properties of nanofluidics devices. Even without the preset surface charge on the confining walls, as shown in this work, a potential difference between inside and outside nanopores can be established based on hydration and interfacial effects with non-electrostatic interactions. Substantial charge neutrality breakdown occurs inside nanopores and charge balance is only maintained when ionic charges inside and outside nanopores are included. This is also reflected by the nanopore model used in this work that is distinct from the conventional way of describing charge distribution inside nanopores in two key aspects, one is the inclusion of non-electrostatic interactions and the other is solving the charge distributions inside and outside the nanopore simultaneously with no preset boundary conditions (a given surface potential or a preset surface charge density). To summarize, we employed quantitative NMR measurements and numerical calculations on a new nanopore model to investigate the electroneutrality condition in nanoconfined aqueous electrolytes. Substantial electroneutrality breakdown of the total charge is observed inside uncharged activated carbon nanopores. The ion-specific interfacial interactions and ion–ion correlations are found to play critical roles in determining the extent of the electroneutrality breakdown. These effects are further investigated in charged carbon nanopores, which lead to strong asymmetric responses of cations and anions to the confining wall surface charging. Moreover, anions impose great influence on the cation’s behaviour via the ion–ion correlations. Our study demonstrates that graphitic-like porous carbon provides an ideal model system, and that the novel in situ NMR approach opens a new avenue for quantitative experimental evaluations of various ion-specific interactions near the interface and under nanoconfinement. Although our work is based on aqueous electrolytes, it can be generally applied to other systems such as organic electrolyte and ionic liquids where the strong ion-specific properties beyond their electrovalencies (for example, ion solvation, interaction with the surface, ion–ion correlations) are also of relevance. The NMR approach is also of great value for validating theories [36] , [55] , [56] where the possibility of nanoconfinement-induced electrolyte non-neutrality in aqueous electrolytes is often ignored in computational studies, which commonly assume a priori a neutrality of the total charge in nanoconfined regions. The findings revealed by the NMR study have broad implications because the electroneutrality breakdown in aqueous electrolytes can be very substantial in nanoconfined regions, which exist in many systems including proteins, desalination devices, colloidal suspensions and supercapacitors. Carbon material P-40 preparation Porous carbon used in this work is derived from high-temperature PEEK using a procedure modified from previous reports [17] , [22] . PEEK pellets are carbonized at 900 °C for 30 min in Argon atmosphere. The carbonized chunk is then cooled down to room temperature and subsequently ground into small particles of ~0.5 mm in diameter. The pulverized sample is activated at 900 °C under water vapour for a designated time to achieve certain burn-off percentage. The pulverization ensures uniform activation, which leads to a narrow pore size distribution. The mass reduction achieved by the activation process is 40% and the corresponding sample is designated as P-40. The average pore size of P-40 is 0.9 nm from wall surface to wall surface assuming a slit-shaped pore (1.2 nm from carbon centre to carbon centre) according to the previous study [17] . The sample that has undergone a mass reduction of 92% during the activation process is labelled as P-92, whose pore size is 1.9 nm (carbon to carbon centres). Nanoconfined electrolytes preparation The sodium salts are purchased from Sigma-Aldrich and used as purchased without further purification. The purity is >99.0% expect for NaBF 4 (>98%). The aqueous electrolytes are prepared to contain Na + cations 1 mol kg −1 except for NaF (0.8 mol kg −1 because of its lower solubility in water). A simple procedure is followed for preparing the nanoconfined aqueous electrolyte. In general, 30 μl electrolyte is injected into 20 mg P-40 sample. The mixture is then tightly sealed in an NMR sample tube. P-40 has a pore volume of 0.5 cm 3 g −1 therefore 30 μl electrolyte is sufficient to fill the nanopore and about two thirds of the electrolyte is left in the intergranular space. Device to control carbon surface charging The device used to control carbon surface charging is comprised of two electrodes made of pure P-40 separated by a glass fibre and immersed in the aqueous electrolyte (1 mol kg −1 NaBF 4 or NaNO 3 ). Each electrode is 3 mm long and 2.5 mm in diameter. One electrode is shielded with a copper foil so that the detected NMR signal comes only from a single electrode. Potential is applied between the two electrodes. The charging process is similar to a supercapacitor. In brief, cations are driven away from the surface and anions are attracted to the surface of positive charging such that the net charge on the electrolyte side balances the electric charge on the carbon surface. Static NMR on uncharged P-40 1 H, 23 Na, 19 F (for NaF and NaBF 4 ) and 15 N (for NaNO 3 , 15 N enriched) static spectra on the electrolyte/P-40 mixture are measured with a 400 MHz pulsed NMR system at 293 K. A single-pulse sequence is used for measurement and the last delay is set long enough to make sure the signal is fully recovered after each scan. Free induction decay data acquisition starts at 5 μs (ring-down time) after the 90° pulse. The spectral linewidth of full-width at half-maximum is ~5 p.p.m. for all the nuclei determined by susceptibility anisotropy broadening. Since the peak widths associated with nuclei inside and outside pores are very similar, the effect will not cause biased estimate of the ratio between the peak intensity for ions inside nanopores versus that outside nanopores. It is this ratio that was used to calculate the ion concentrations. is about 160 μs for 19 F and about 640 μs for 23 Na. These are much longer than 5 μs and the intensity decay over 5 μs is insignificant. It was found that extrapolating the free induction decay intensity back to t =0 exponentially does not change the determination of the ion concentrations. The 90° pulse of Na + inside P-40 nanopores is shown to be the same as Na + in the intergranular space as well as in pure aqueous electrolyte solution. Furthermore, there are no sidebands under 7 kHz magic angle spinning. All these indicate that the quadrupole interaction effect is negligible for 23 Na NMR. Ion concentration calculation The two peaks in the 23 Na NMR spectrum (representing ions in the nanopores and ions in the intergranular space) are well separated and are deconvoluted to obtain the intensities A in (inside nanopores) and A out (outside nanopores). Since the total number of Na + cations n tot associated with the entire NMR spectrum is known based on the amount of the injected electrolyte, the portion inside P-40 nanopores could be calculated by . Using the same procedure the amounts of water inside and outside nanopores can be determined. From these numbers we can calculate the Na + concentration c inside the P-40 nanopores. The concentrations of BF 4 − and NO 3 − inside and outside nanopores can be determined similarly. In situ NMR on charged P-40 In situ 19 F, 23 Na NMR experiment is carried out on a homemade probe that is equipped with a charging system controlled by Labview. The device to control P-40 surface charging is charged from 0 to 1.0 V with a step of 0.1 V. Static NMR spectrum is acquired when the charging reaches equilibrium, typically after 2 h. For 19 F NMR, the last delay is 5 s and the spin-lattice relaxation time ( T 1 ) is 0.7 s. For 23 Na, the last delay is 0.5 s and T 1 is 20 ms. Charging has little effect on the T 1 relaxation times, , and the 90° pulses for both 19 F and 23 Na. Quadrupole interaction effect for 23 Na is confirmed to be negligible. Numerical calculation The nanopore confinement model is illustrated in Fig. 3a . Two conducting metal plates are immersed in 1 mol l −1 symmetric monovalent electrolyte to simulate the 1D planar carbon nanopore with pore size d . Water is assumed to be a continuum with a dielectric constant ε =78.5. x 1 and x 2 are the ion locations closest to the inner surface and the outer surface respectively, that is, the Helmholtz plane. The cutoff distance x min that an ion can approach the surface is limited by the finite ion size. Here we use the typical hydrated ion radii [57] 0.35 nm as x min for both cations and anions. Using different cutoff distances for cations and anions will only affect the numerical values of the ion concentrations but does not change the electroneutrality breakdown and its dependence on B − . The effect of a smaller cutoff distance for anions on the ion concentration in nanopores is equivalent to increasing the anion propensity for the surface. Therefore without losing generality, we use the same cutoff distances for both ions and change only the B − values to investigate the effects of ion-specific interactions with the surface. The electrostatic potential near the solid–liquid interface is described by the generalized Poisson–Boltzmann equation: Since the system is symmetric with respect to the centre of the pore, designated as x =0, we only need to consider the half space x >0. In the bulk electrolyte side, the ions only experience surface interactions from one side thus , whereas inside the nanopore, ions experience interactions from both the surfaces such that The region between the Helmholtz plane and the metal surface is modelled as a parallel plate capacitor with capacitance C H . This is required for solving the potentials both inside and outside the nanopore simultaneously. The Helmholtz capacitance C H is usually calculated by , giving rise to a capacitance value of 200 μF cm −2 if the dielectric constant of bulk water is used. A smaller capacitance is obtained if reduced dielectric constant is invoked considering the dipole saturation at the interface [34] , [58] . Instead of using a smaller value for C H , here we adopt a larger value C H =400 μF cm −2 for the metal surface to emphasize another mechanism that is proposed only recently [59] , [60] . In brief, ions bind to the metal surface via attractions with its image charge and form ion-image dipoles. The capacitance can be very large because external charging is mainly to overcome the weak dipole–dipole repulsion between the bound ions. The unique solution of the electrostatic potential ψ ( x ) for the half space x> 0 is determined using two boundary conditions: (1) electrostatic potential in the bulk electrolyte is 0, that is, ψ (∞)=0; (2) in the pore centre and two constraints: (3) the total electrolyte charge inside the nanopore is balanced by the total electrolyte charge outside the nanopore (equivalently the metal plate can carry induced charge on both the inner surface and the outer surface but the net charge remains 0); (4) the metal plate has equal potential on the inner surface and the outer surface (equivalently the potential drop between the Helmholtz planes at the two sides of the metal plate is , where σ is the total electrolyte charge inside the nanopore). How to cite this article: Luo, Z.-X. et al . Electroneutrality breakdown and specific ion effects in nanoconfined aqueous electrolytes observed by NMR. Nat. Commun. 6:6358 doi: 10.1038/ncomms7358 (2015).